Ultra-stable and highly reactive colloidal gold nanoparticle catalysts protected using multi-dentate metal oxide nanoclusters Owing to their remarkable properties, gold nanoparticles are applied in diverse fields, including catalysis, electronics, energy conversion and sensors. However, for catalytic applications of colloidal gold nanoparticles, the trade-off between their reactivity and stability is a significant concern. Here we report a universal approach for preparing stable and reactive colloidal small (~3 nm) gold nanoparticles by using multi-dentate polyoxometalates as protecting agents in non-polar solvents. These nanoparticles exhibit exceptional stability even under conditions of high concentration, long-term storage, heating and addition of bases. Moreover, they display excellent catalytic performance in various oxidation reactions of organic substrates using molecular oxygen as the sole oxidant. Our findings highlight the ability of inorganic multi-dentate ligands with structural stability and robust steric and electronic effects to confer stability and reactivity upon gold nanoparticles. This approach can be extended to prepare metal nanoparticles other than gold, enabling the design of novel nanomaterials with promising applications. Gold nanoparticles have been the subject of extensive investigation in recent decades because of their exceptional reactivity and broad applicability in various research fields, including catalysis, energy conversion, medicine, electronics, optics, magnetic materials and sensors [1] , [2] , [3] , [4] , [5] , [6] , [7] , [8] . Owing to their large surface area and abundant surface active sites, small gold nanoparticles exhibit high reactivity, which renders them particularly attractive for catalytic applications [1] , [2] , [3] , [4] , [5] , [6] . In this context, intense research attention has been devoted to the development of supported gold nanoparticles to address their inherent instability in past decades; however, the complexity in determining the reactive sites and the difficulty in realising fine-tuning catalysis are critical issues that appear during their applications [1] , [2] , [3] , [4] . Hence, exploring gold nanoparticles without supports, which are often called colloidal gold nanoparticles, has become an important avenue towards achieving distinct performance in fine-tuning catalysis [2] , [3] , [5] , [9] . 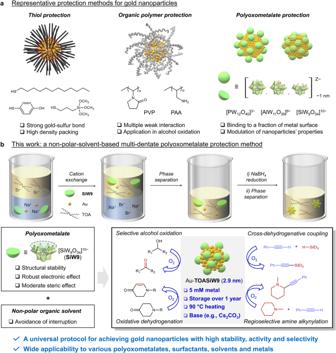Fig. 1: Preparation of gold nanoparticles. aRepresentative methods for the preparation of gold nanoparticles using thiol protection, organic polymer protection and polyoxometalate protection.bThis work: a non-polar-solvent-based multi-dentate polyoxometalate protection method for developing ultra-stable and highly reactive gold nanoparticle catalysts (TOA tetraoctylammonium). To stabilise reactive gold nanoparticles in solutions, various chemicals have been employed as protecting agents, such as citric acid, alkanethiols, amines, surfactants and organic polymers (Supplementary Table 1 , Entries 1–12) [9] , [10] , [11] , [12] , [13] , [14] , [15] , [16] , [17] . In particular, the introduction of the use of alkanethiols constituted an important breakthrough in the development of small (1–3 nm) gold nanoparticles with long-term (months) stability based on the strong affinity of alkanethiols to gold nanoparticles (Fig. 1a ) [10] , [11] . However, the stability of these gold nanoparticles comes at the expense of their reactivity due to reserved surface active sites and high ligand packing density, which hinder substrate access [9] , [12] , [13] . Meanwhile, although organic polymers such as polyvinylpyrrolidone (PVP) are used to prepare gold nanoparticles that perform in alcohol oxidation reactions, their applicability in catalytic reactions requires further validation (Fig. 1a ) [17] . Another concern is that organic protecting agents can react under catalytic conditions, undergoing structural changes and/or detaching from gold nanoparticles during use, leading to destabilisation [12] , [13] , [14] , [15] , [16] . Therefore, the development of a universal methodology for obtaining stable colloidal gold nanoparticles while maintaining high reactivity for various catalytic reactions is an important yet challenging task. Fig. 1: Preparation of gold nanoparticles. a Representative methods for the preparation of gold nanoparticles using thiol protection, organic polymer protection and polyoxometalate protection. b This work: a non-polar-solvent-based multi-dentate polyoxometalate protection method for developing ultra-stable and highly reactive gold nanoparticle catalysts (TOA tetraoctylammonium). Full size image Metal oxide supports have occupied a central role in the field of metal nanoparticle catalysts owing to their ability to enhance the stability of gold and other metal nanoparticles, control their electronic states and achieve synergistic effects [3] , [4] , [6] , [18] . In this regard, polyoxometalates (POMs), a type of anionic metal oxide nanoclusters with diverse properties and functionalities [19] , [20] , [21] , [22] , [23] , [24] , [25] , [26] , have emerged as efficient protecting agents for stabilising metal nanoparticles by means of efficient coordination, electrostatic repulsion and steric hindrance (Fig. 1a and Supplementary Table 1 , Entries 13 − 24) [27] , [28] , [29] , [30] , [31] , [32] , [33] , [34] , [35] , [36] , [37] . In addition to an exceptional steric effect, owing to which bulky POM ligands only bind to a fraction of the metal surface, thus ensuring substrate access, the adaptable structures and properties of functional POM ligands enable a molecular-level catalyst design for achieving fine-tuning catalysis and synergistic effects [33] , [34] , [35] , [36] . However, POM-protected gold nanoparticles sometimes undergo agglomeration in solution during storage and/or usage [31] , [32] , [36] , [37] , which can be attributed to decomposition and structure transformation of POMs in the commonly used aqueous media or occupation of the vacant sites of POMs by alkali metal cations and solvent molecules, leading to destabilization of gold nanoparticles [38] , [39] , [40] , [41] . Moreover, the restriction to hydrophilic use besides the semi-stability issue of POM-protected gold nanoparticles has also limited the exploration of such a feasible molecular-level catalyst design towards practical catalytic applications [32] . Accordingly, we recently applied utilisation of POMs to design various metal oxo clusters and metal clusters in organic solvents, where we have shown that the above-mentioned troubles in aqueous media can be avoided [42] , [43] , [44] . Here we present a feasible method for obtaining ultra-stable and highly reactive small gold nanoparticles (of ~3 nm) by employing multi-dentate POM ligands in a non-polar solvent system (e.g. toluene, Fig. 1b ). Notably, the resultant small gold nanoparticles exhibit exceptional high stability in solution even under harsh conditions such as high concentration (>5 mM metal), long-term storing (>1 year), heating (~90 °C) and addition of bases (e.g. K 2 CO 3 and Cs 2 CO 3 ), which are typically required in catalytic applications. These POM-stabilised gold nanoparticles exhibit high catalytic performance in the aerobic oxidation of alcohols with wide substrate scope and high selectivity to aldehyde or ketone products without changes in the particle size. Additionally, these colloidal gold nanoparticles are effective for various catalytic oxidation reactions using molecular oxygen (O 2 ) as the sole oxidant. This methodology can be extended to various POM ligands, metals (e.g. platinum, ruthenium, rhenium and rhodium) and solvent systems (e.g. p -xylene and 1,2-dichloroethane) to produce small metal nanoparticles stabilised by multi-dentate POM ligands, which demonstrates its wide applicability and versatility. Development of a non-polar-solvent-based multi-dentate POM protection method Gold nanoparticles protected by multi-dentate [SiW 9 O 34 ] 10− ( SiW9 ) ligands in toluene (Au- TOASiW9 ) were prepared according to the following method (Fig. 1b ): first, separate aqueous solutions of chloroauric acid (HAuCl 4 ) and the sodium salt of SiW9 ( NaSiW9 ) were prepared and transferred into toluene using tetraoctylammonium bromide (TOAB) as a phase transfer agent. Afterwards, an aqueous solution of sodium borohydride (NaBH 4 ) was slowly added to the resulting solution leading to a fast colour change in the toluene phase from orange to dark red (Supplementary Fig. 1 ), followed by a phase separation process to yield toluene solution of Au- TOASiW9 . A characteristic surface plasmon resonance band attributed to the gold nanoparticles of Au- TOASiW9 was observed at 524 nm in the ultraviolet–visible (UV–vis) spectrum (Supplementary Fig. 2 ). It should be noted that an excess amount of TOAB and a minimal amount of NaBH 4 are required; the former facilitates the transfer of SiW9 as ligands into the toluene phase until reaching the cation exchange equilibrium (Supplementary Fig. 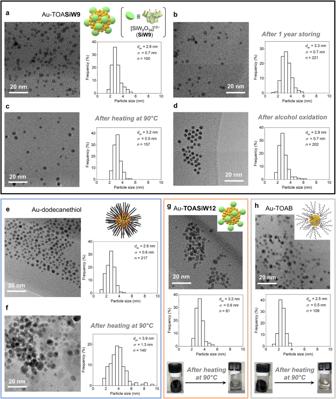Fig. 2: Characterisation and stability test of gold nanoparticles. TEM images and size distribution histograms:aAu-TOASiW9.bAu-TOASiW9after storing for 1 year.cAu-TOASiW9after heating at 90 °C for 24 h.dAu-TOASiW9after alcohol oxidation in the presence of Cs2CO3under the conditions shown in Table1, entry 2.eAu-dodecanethiol.fAu-dodecanethiol after heating at 90 °C for 24 h.gAu-TOASiW12(the bottom picture shows the formation of precipitates from Au-TOASiW12after heating at 90 °C for 24 h).hAu-TOAB (the bottom picture shows the formation of precipitates from Au-TOAB after heating at 90 °C for 24 h). 3 ) and the latter prevents the reverse transfer of TOASiW9 into the aqueous phase, in which 10 equivalents of TOAB and 4 equivalents of NaBH 4 relative to HAuCl 4 were found to be the optimal conditions (Supplementary Table 2 ). Transmission electron microscopy (TEM) observation of Au -TOASiW9 indicated an average particle size (2.9 nm) comparable to that of dodecanethiol-protected gold nanoparticles (Au-dodecanethiol, 2.6 nm), which were synthesised via the classic Brust–Schiffrin method for comparative purposes (Fig. 2a, e ) [10] . Additionally, gold nanoparticles protected only by the surfactant TOAB (Au-TOAB, 2.5 nm) and fully occupied POM [SiW 12 O 40 ] 4− (Au- TOASiW12 , 3.2 nm) were also prepared (Fig. 2g, h ). Fig. 2: Characterisation and stability test of gold nanoparticles. TEM images and size distribution histograms: a Au- TOASiW9 . b Au- TOASiW9 after storing for 1 year. c Au- TOASiW9 after heating at 90 °C for 24 h. d Au- TOASiW9 after alcohol oxidation in the presence of Cs 2 CO 3 under the conditions shown in Table 1 , entry 2. e Au-dodecanethiol. f Au-dodecanethiol after heating at 90 °C for 24 h. g Au- TOASiW12 (the bottom picture shows the formation of precipitates from Au- TOASiW12 after heating at 90 °C for 24 h). h Au-TOAB (the bottom picture shows the formation of precipitates from Au-TOAB after heating at 90 °C for 24 h). Full size image Generally, colloidal gold nanoparticles suffer from stability issues such as concentration limitation due to the salting-out effect and agglomeration during use [2] , [5] , [9] , [12] . In contrast, this methodology allows employing metal precursors at concentrations exceeding 5 mM, which are significantly higher than those used in previously reported methods (Supplementary Table 1 , Entries 13 − 25). The stability of the small (~3 nm) gold nanoparticles prepared in this study was evaluated under long-term storage, heating treatment and addition of bases, which are general requirements for practical catalytic applications in solution [1] , [2] , [3] , [4] , [5] , [6] , [12] , [13] , [14] , [15] . Au- TOASiW9 exhibited exceptional stability, retaining its particle size and size distribution during storage in toluene at room temperature (~25 °C) for over 1 year (Fig. 2b ). In contrast, Au-TOAB underwent agglomeration within 2 months (Supplementary Fig. 4 ). Additionally, Au- TOASiW9 displayed an extraordinary stability under heating conditions, maintaining its particle size after continuous stirring at 90 °C for 24 h, whereas the particle size of Au-dodecanethiol increased, and Au-TOAB and Au- TOASiW12 agglomerated and precipitated under the same conditions (Fig. 2c, f–h ). Au- TOASiW9 also showed strong resistance to the addition of bases such as Cs 2 CO 3 , whereas Au-TOAB and Au-dodecanethiol agglomerated and partially precipitated under the same conditions (Supplementary Fig. 5 ). The precipitation of Au-dodecanethiol can be ascribed to the oxidation of thiol ligands to disulfides followed by detachment from the gold nanoparticles [14] , which highlights the stability issue of the ligands themselves during use. Notably, even after participating in catalytic aerobic alcohol oxidations in the presence of a base, Au- TOASiW9 retained its particle size and size distribution (see Fig. 2d and subsequent discussion). Taken together, these results indicate that Au- TOASiW9 is much more stable than the well-known Au-dodecanethiol and exhibits resistance to heating and addition of bases, which are essential conditions in catalysis, and multi-dentate POM ligands are key for achieving high stability. To demonstrate the applicability and versatility of this practical approach, it was successfully expanded to other organic solvents, such as p- xylene and 1,2-dichloroethane, and to various types of POMs, including trivacant SiW9 , fully occupied SiW12 , monovacant [SiW 11 O 39 ] 8− ( SiW11 ) and divacant [SiW 10 O 36 ] 8− ( SiW10 ), furnishing small (~3 nm) gold nanoparticles under similar synthetic conditions (Supplementary Fig. 6 ). Furthermore, small nanoparticles (<5 nm) of different metals, including platinum, ruthenium, rhenium and rhodium were successfully synthesised (Supplementary Fig. 7 ). Next, zeta potential measurements were performed to investigate the surface state of the gold nanoparticles (Fig. 3a ). The observed negative zeta potential for the POM-protected gold nanoparticles indicated the formation of anionic POM layers surrounding the gold nanoparticles [31] , [32] , [33] . Au- TOASiW9 exhibited the most negative zeta potential, suggesting the strongest interparticle electrostatic repulsion that effectively prevents agglomeration. The aberration-corrected annular dark-field scanning TEM (ADF-STEM) images of Au- TOASiW9 showed the presence of shells on the surface of the gold nanoparticles (Fig. 3b , Supplementary Fig. 8 ), and elemental mapping using energy-dispersive X-ray spectroscopy (EDS) further confirmed the formation of an Au-core–POM-shell-like structure (Fig. 3c ). Through titration experiments of dodecanethiol to Au- TOASiW9 with inspiration by previous reports [29] , [30] , it was estimated that around 30 SiW9 ligands surrounded a 3 nm gold particle, and surface coverage can be estimated as 47% (Supplementary Fig. 9 , see explanation in detail). Subsequently, X-ray photoemission spectroscopy (XPS) showed that the binding energy of the Au 4 f 7/2 region of Au- TOASiW9 (82.3 eV) was notably lower than that of bulk Au (84.0 eV) and Au-TOAB without POM protection (83.2 eV, Fig. 3d , Supplementary Fig. 10 ), indicating the anionic status of the POM-protected gold nanoparticles stemming from the electronic interaction between anionic POM ligands and gold nanoparticles [31] , [32] , [33] , [34] , [35] , [36] . Notably, the binding energy of Au- TOASiW9 (82.3 eV) was even lower than those of reported anionic gold nanoparticles, PVP-protected gold nanoparticles (Au:PVP, 82.7 eV) and SiW11 -protected gold nanoparticles (82.8 eV), which were obtained in aqueous solution [17] , [33] . No obvious difference in the binding energies was found between Au- TOASiW12 and Au-TOAB, highlighting the importance of a robust electronic interaction between multi-dentate POM ligands and gold nanoparticles in this system. Moreover, POM-protected gold nanoparticles with similar particle sizes possessed sequentially modulated electronic states (Fig. 3d ), providing a feasible and effective tool for adjusting the activity of gold nanoparticle catalysts, as previously discussed in detail [36] . Fig. 3: Investigations of the structure and electronic state of Au-TOASiW9. a Zeta potential of Au- TOASiW9 , Au- TOASiW10 , Au- TOASiW11 , Au- TOASiW12 , Au-TOAB and Au-dodecanethiol in toluene. b Representative atomic-resolution annular dark field scanning transmission electron microscopy (ADF-STEM) image of Au- TOASiW9 . c EDS elemental mapping images of Au- TOASiW9 . d XPS spectra of various ligand-protected gold nanoparticles and bulk Au (the arrow indicates the trend of changes in binding energy). e W L 3 -edge XANES spectra with associated second derivatives of TOASiW9 and Au- TOASiW9 . f k 3 -Weighted W L 3 -edge EXAFS spectra of TOASiW9 and Au- TOASiW9 . g , Relative energy of SiW9 -protected gold nanoparticles and models of the optimised structures for different orientations of SiW9 . Full size image To confirm the structures of the POM ligands after hybridisation with gold nanoparticles, solid samples of TOASiW9 and Au- TOASiW9 obtained by evaporating the toluene solvent were characterised. Infra-red (IR) spectroscopies showed that Au- TOASiW9 exhibited similar bands to those of TOASiW9 and NaSiW9 regarding characteristic peaks in the region from 800 to 1000 cm −1 , but differed from those of sodium tungstate, indicating that the structure of SiW9 was preserved (Supplementary Fig. 11 ) [34] , [36] . According to Raman spectroscopies, the characteristic peak of W=O d bonding from POM structures was observed at 965 cm −1 for Au- TOASiW9 and TOASiW9 , similar to that of the tetrabutylammonium salt of SiW9 (TBA 4 H 6 SiW 9 O 34 , TBASiW9 ) at 970 cm −1 but slightly shifted from that of the sodium salt of SiW9 (Na 10 SiW 9 O 34 , NaSiW9 ) at 940 cm −1 (Supplementary Fig. 12 ). This can be ascribed to the presence of sodium cations near the POM anions in the case of NaSiW9 increasing the W=O bonding length and weakening the bonding strength [45] . To analyse the precise POM structure, X-ray absorption fine structure analyses were conducted. Similar patterns of Au- TOASiW9 and TOASiW9 in the second derivative of white-line region and W L 3 -edge k -space EXAFS spectra, indicating that POMs maintained their structures after hybridization with gold nanoparticles (Fig. 3e, f ) [36] , [46] . Then, similar patterns of TOASiW9 and NaSiW9 but completely different from those of the potassium salt of SiW12 (K 4 SiW 12 O 40 , KSiW12 ) and WO 3 in the second derivative of white-line region indicated that there existed no obvious structural changes in the {WO 6 } octahedra (Supplementary Fig. 13a, b ). The W L 3 -edge k -space EXAFS spectra showed no significant changes between TOASiW9 and NaSiW9 while in contrast to that of KSiW12 and WO 3 , strongly indicating that POM maintained intact structures as well (Supplementary Fig. 13c ). In the R- space EXAFS spectra, the peaks at R = 1.2, 1.7 and 3.2 Å assignable to terminal W=O, bridging W−O−W and W−W, respectively, exhibited no drastic changes from NaSiW9 to TOASiW9 , further supporting the preservation of POM structures in this method (Supplementary Fig. 13d ). Finally, structures of POMs during synthesis of gold nanoparticles were confirmed through deliberately transferring them into aqueous phase (Supplementary Fig. 14 , Supplementary Table 2 , Entry 5). In the IR spectra, the characteristic peaks of SiW9 in the region of 500 − 1000 cm −1 were well consistent between NaSiW9 and POMs after mixing with gold precursors and sodium borohydride respectively, indicating their intact structures in current method (Supplementary Fig. 14 ). These results demonstrate that POM ligands remain stable in this synthetic system, effectively protecting the metal nanoparticles. The interaction between SiW9 and gold nanoparticles was further investigated by performing first-principles calculations. Considering that the interaction of bulky tetraoctylammonium (TOA) cations and toluene solvent molecules with POMs was negligible, structural optimisations were conducted using one multi-dentate SiW9 ligand with several different orientations on the surface of 2-nm-large gold nanoparticle without TOA cations and solvent molecules (Fig. 3g ). The most stable orientation was identified as that in which multi-dentate SiW9 interacted with a gold nanoparticle at the vacant site of SiW9 . These results demonstrate that the coordination of gold nanoparticles at the vacant sites of SiW9 effectively contributes to the nanoparticle stabilisation and, together with the experimental results, highlighting the essential role of an adequate coordination of POM ligands in protecting metal nanoparticles during synthesis, storage and use. Hence, the development of ultra-stable small metal nanoparticles via POM protection was successfully achieved in a non-polar solvent for the first time (Fig. 1b ). Oxidation reactions catalysed by ultra-stable small gold nanoparticles The high concentration and extraordinary stability of the developed colloidal gold nanoparticles even under heating conditions and in the presence of bases prompted us to explore their performance in liquid-phase catalytic reactions. Anionic gold nanoparticles have been proved effective in activating O 2 , which renders them potential catalysts in aerobic oxidation reactions; however, only a few studies have been conducted so far [17] , [33] , [36] . Therefore, the low binding energy of the Au 4 f 7/2 region of Au- TOASiW9 motivated us to investigate the catalytic performance for various aerobic oxidation reactions in solution, particularly those requiring heating treatment or addition of bases, starting with aerobic alcohol oxidation as a typical model reaction of gold nanoparticle catalysts. 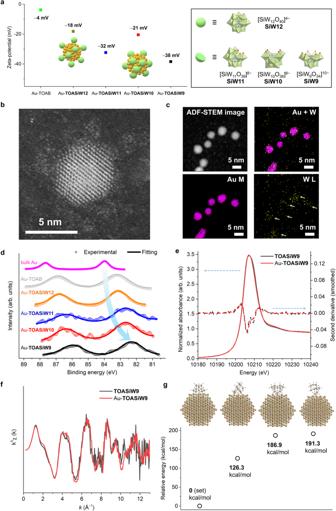Fig. 3: Investigations of the structure and electronic state of Au-TOASiW9. aZeta potential of Au-TOASiW9, Au-TOASiW10, Au-TOASiW11, Au-TOASiW12, Au-TOAB and Au-dodecanethiol in toluene.bRepresentative atomic-resolution annular dark field scanning transmission electron microscopy (ADF-STEM) image of Au-TOASiW9.cEDS elemental mapping images of Au-TOASiW9.dXPS spectra of various ligand-protected gold nanoparticles and bulk Au (the arrow indicates the trend of changes in binding energy).eW L3-edge XANES spectra with associated second derivatives ofTOASiW9and Au-TOASiW9.fk3-Weighted W L3-edge EXAFS spectra ofTOASiW9and Au-TOASiW9.g, Relative energy ofSiW9-protected gold nanoparticles and models of the optimised structures for different orientations ofSiW9. 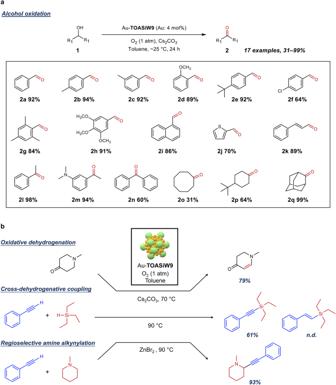Fig. 4: Reaction scope. aSubstrate scope of Au-TOASiW9-catalysed aerobic alcohol oxidation. Reaction conditions: alcohol (0.25 mmol), 3 mL toluene solution of Au-TOASiW9(Au: 4 mol%), Cs2CO3(0.5 mmol), ~25 °C (room temperature), O2(1 atm), 24 h.bSchematic of various aerobic oxidation reactions catalysed by Au-TOASiW9. Detailed reaction conditions are described in Method section. Among the examined POM-protected gold nanoparticle catalysts, Au- TOASiW9 exhibited the highest activity towards the aerobic oxidation of benzyl alcohol ( 1a ) in the presence of K 2 CO 3 as a base to selectively furnish benzaldehyde ( 2a ) as a product (Table 1 and Supplementary Table 3 ). A sequentially modulated activity was found depending on the type of POM in line with the electronic states of gold nanoparticles, which can be correlated with the effective activation of O 2 on anionic gold nanoparticles (Table 1 , Entries 1–5; Fig. 3d and Supplementary Fig. 15 ). In contrast, gold nanoparticles including Au- TOASiW12 , Au-TOAB and Au-dodecanethiol exhibited significantly low catalytic activity (Fig. 1a ; Table 1 , Entries 5–7). Notably, no significant changes were observed in the particle size of the gold nanoparticles protected with SiW9 , SiW10 and SiW11 even after the reaction, and no significant decrease was observed in the catalytic activity of Au- TOASiW9 during the reaction (Supplementary Figs. 16 and 17 ). Furthermore, Raman spectra showed that Au- TOASiW9 after the catalytic oxidation of 1a exhibited similar characteristic bands with Au- TOASiW9 , indicating that the structure of SiW9 was preserved (Supplementary Fig. 12 ). In contrast, an evident agglomeration of gold nanoparticles was observed during the reaction using fully occupied SiW12 as a protecting ligand (Supplementary Fig 17 ). These results indicated that the presence of vacant (coordination) sites in the POM ligands is essential for protecting the metal nanoparticles. Nevertheless, Au-TOAB underwent more severe agglomeration than Au- TOASiW12 , indicating that POM ligands can generally function as stabilising agents in comparison to conventional organic substances [31] , [32] . Considering that the particle size of Au-dodecanethiol was kept after the reaction (Table 1 , Entry 7; Supplementary Fig. 17 ), its low catalytic activity was likely due to difficulties in substrate access and strong bonding of thiol ligands to the surface of gold nanoparticles [12] , [13] . Meanwhile, Au- TOASiW9 exhibited higher catalytic activity when using Cs 2 CO 3 as a base than in the presence of K 2 CO 3 , and 2a was still selectively produced from 1a while maintaining the small particle size (Table 1 , Entry 2; Fig. 2d ). In contrast, the reaction barely proceeded using Au-dodecanethiol and Cs 2 CO 3 due to the oxidation of the thiol ligands, which led to precipitation of gold nanoparticles (Table 1 , Entry 8) [14] . Table 1 Selective aerobic oxidation of benzyl alcohol (1a) to benzaldehyde (2a) a Full size table Additionally, TOASiW9 exhibited no activity and Au- TOASiW9 did not promote the reaction under argon (Ar) atmosphere, confirming gold nanoparticles as the active sites and O 2 as the terminal oxidant in this catalysis (Table 1 , Entries 9 and 10). The kinetic isotope effect (KIE) was then examined for Au- TOASiW9 -catalysed oxidation of 1a . Under O 2 atmosphere (1 atm), a much higher reaction rate was observed for 1a than benzyl-α,α- d 2 alcohol ( k H / k D = 3.2, Supplementary Fig. 18 ), indicating that C−H cleavage can be the turnover limiting step. When the reaction was carried out under air atmosphere (O 2 , 0.2 atm), no significant KIE was observed ( k H / k D = 1.2, Supplementary Fig. 19 ), suggesting that O 2 adsorption and/or activation can be turnover limiting step under air atmosphere (Supplementary Fig. 15 ). To investigate the effect of cations, preparation of gold nanoparticles protected with SiW9 was examined using different cations such as tetrahexylammonium (THA), tetradecylammonium (TDA), and cetyltrimethylammonium (CTA) instead of TOA. Although TDA can be used for preparation of gold nanoparticles, incomplete phase transfer was observed for THA and CTA owing to less hydrophobicity of metal precursors and emulsion formation, respectively (Supplementary Fig. 20a ). The obtained gold nanoparticles using TDA cations and SiW9 (Au- TDASiW9 ) possessed similar particle sizes of 3 nm and similar catalytic reactivity to those of Au- TOASiW9 , suggesting that countercations did not necessarily facilitate the reaction (Supplementary Fig. 20b, c ). These results provide direct evidence that multi-dentate POM ligands do not only contribute to stabilising the small (~3 nm) gold nanoparticles during their preparation but also allow retaining their catalytically active sites, enabling the modulation of the electronic states of gold nanoparticles for activity control. Furthermore, the Au- TOASiW9 -catalysed reaction demonstrated a broad substrate scope, enabling the conversion of various primary and secondary alcohols to the corresponding aldehyde and ketone products, respectively (Fig. 4a , Supplementary Fig. 21 ). When Cs 2 CO 3 was used as a base at room temperature (~25 °C), Au- TOASiW9 efficiently promoted the oxidation of benzyl alcohol as well as benzylic alcohols with either electron-withdrawing or electron-donating groups, affording the corresponding benzaldehydes ( 2a – 2i ). Au- TOASiW9 successfully catalysed the oxidation of a heteroaromatic alcohol to the corresponding aldehyde ( 2j ). In addition, an α,β-unsaturated alcohol afforded the corresponding α,β-unsaturated aldehyde ( 2k ), and aromatic and aliphatic secondary alcohols also gave the corresponding ketones ( 2l – 2q ). Fig. 4: Reaction scope. a Substrate scope of Au- TOASiW9 -catalysed aerobic alcohol oxidation. Reaction conditions: alcohol (0.25 mmol), 3 mL toluene solution of Au- TOASiW9 (Au: 4 mol%), Cs 2 CO 3 (0.5 mmol), ~25 °C (room temperature), O 2 (1 atm), 24 h. b Schematic of various aerobic oxidation reactions catalysed by Au- TOASiW9 . Detailed reaction conditions are described in Method section. Full size image Finally, the applicability of Au- TOASiW9 towards various oxidation reactions using O 2 as the sole oxidant was confirmed (Fig. 4b , Supplementary Fig. 22 ). In addition to the high reactivity and wide applicability in alcohol oxidation reactions, Au- TOASiW9 catalysed the oxidative dehydrogenation of N -methyl piperidone in toluene in the presence of Cs 2 CO 3 as a base (Supplementary Fig. 23a ). Subsequently, the cross-dehydrogenative coupling (CDC) reaction of a terminal alkyne and a hydrosilane in the presence of O 2 as the hydrogen acceptor efficiently proceeded using Au- TOASiW9 to afford the desired alkynylsilane without formation of hydrosilylation products. In contrast, when the CDC reaction was performed under the same conditions using typical supported gold nanoparticle catalysts, the undesirable hydrosilylation reaction occurred to a certain extent (Supplementary Fig. 23b ) [47] . The observed high selectivity to the CDC product when using Au- TOASiW9 can be attributed to a fast Au–hydride oxidation induced by activated oxygen species on the anionic gold nanoparticles preventing the hydrosilylation reaction. Moreover, in a regioselective alkynylation of a tertiary amine, Au -TOASiW9 demonstrated comparable reactivity to the reported catalytic system using supported gold nanoparticles in the presence of ZnBr 2 (Supplementary Fig. 22c ) [48] . These findings demonstrate that this methodology provides a universal protocol for the preparation of colloidal metal nanoparticle catalysts simultaneously exhibiting high reactivity, stability and selectivity that can compete with conventional supported metal nanoparticle catalysts. In summary, we have developed a non-polar-solvent-based multi-dentate POM protection strategy for obtaining ultra-stable and catalytically active colloidal gold nanoparticles. These small gold nanoparticles exhibited remarkable tolerance towards high concentration conditions (>5 mM metal), long-term storage (>1 year), heating treatment (>90 °C) and addition of bases (e.g. Cs 2 CO 3 ) without undergoing changes in particle size and size distribution. They exhibited a high reactivity and selectivity in various catalytic oxidation reactions using O 2 as the sole oxidant, including alcohol oxidation, piperidone dehydrogenation, terminal alkyne–hydrosilane cross-dehydrogenative coupling and tertiary amine alkynylation. The robust electronic and moderate steric effects of multi-dentate POM ligands are considered essential to achieve an extraordinary catalytic performance. The wide applicability to various POM ligands, solvent systems and metal nanoparticles, and the broad reaction scope render this approach highly promising for solving the compromise between reactivity and stability of metal-nanoparticle-based materials in diverse fields including catalysis, biochemistry, photochemistry, coordination chemistry, pharmaceuticals, physiochemistry and materials science. Instruments and reagents Gas chromatography (GC) analyses were conducted on Shimadzu GC2014 equipped with a flame ionization detector (FID) and an InertCap-5 capillary column (30 m × 0.25 mm × 0.25 μm) using Shimadzu CR8A Chromatopac Data Processor for area calculations. GC mass spectrometry (GC-MS) analyses were performed by Shimadzu GCMS-QP2020 equipped with an InertCap-5 MS/NP capillary column (30 m × 0.25 mm × 0.25 μm) at an ionization voltage of 70 eV. Inductively coupled plasma atomic emission spectroscopy (ICP-AES) analyses were conducted by Shimadzu ICPS-8100. Transmission electron microscope (TEM) observations were conducted by JEM-2000EX and JEM-2010F at an acceleration voltage of 200 kV, and scanning transmission electron microscopy (STEM) observations were conducted by JEM-ARM200F Thermal FE at an acceleration voltage of 200 kV and JEM-ARM300CF with a cold FE at an acceleration voltage of 300 kV. The illumination semi-angle and the collection semi-angle for atomic-resolution annular dark field (ADF-)STEM images were acquired 30 mrad and 32–200 mrad, respectively. W L 3 -edge X-ray absorption spectroscopy (XAS) was carried out at the BL01B1 beamline of SPring-8. X-ray absorption fine structure (XAFS) measurements were conducted in transmission mode using a Si(111) double-crystal monochromator. The X-ray absorption near-edge structure (XANES) and extended X-ray absorption fine structure (EXAFS) spectra were analysed using xTunes programme [49] . Pre-edge backgrounds were subtracted using a McMaster equation. EXAFS backgrounds were subtracted using a cubic spline method (spline range = 5). W L 3 -edge EXAFS spectra in k -space were obtained as k 3 -weighted χ spectra after normalization. The X-ray photoelectron spectroscopy (XPS) was performed on ULVAC-PHI PHI5000 VersaProbeIII at the Advanced Characterisation Nanotechnology Platform of The University of Tokyo. The samples were embedded in In foil and brought in the introduction chamber. The fitting of experimental data was conducted using a Multipak software (version 9.2.0.5, by Ulvac-phi, inc.) in which the Shirley method was used for the background and a Gauss−Lorentz type function was performed for fitting. The binding energies were calibrated by using the C 1 s signal of C−C bonding at 284.9 eV. Under these conditions, the Au 4 f 7/2 signal of bulk Au (CAS No. 7440-57-5) was located at 84.0 eV. Solution-state ultraviolet–visible (UV–Vis) spectra were measured on JASCO V-770 spectrometer with a 1 cm quartz cell at room temperature (~25 °C). Zeta-potential measurement were conducted on Malvern Zetasizer NanoZS at a backscatter mode and a working voltage of 40 V was adopted. Infra-red (IR) spectra were measured on a JASCO FT/IR-4100 using the attenuated total reflection method. Raman spectra were measured on a JASCO NRS-5100. All chemical reagents were obtained from Tokyo Chemical Industry, Aldrich, Kanto Chemical, or FUJIFILM Wako Pure Chemical (reagent grade) without pretreatment. Inorganic salts of SiW9 , SiW10 , SiW11 , SiW12 ( NaSiW9 , Na 10 SiW 9 O 34 ; K 8 SiW 10 O 36 ; K 8 SiW 11 O 39 ; K 4 SiW 12 O 40 ) and a tetrabutylammonium salt of SiW9 ( TBASiW9 , (C 16 H 36 N) 4 H 6 SiW 9 O 34 ) were prepared according to the reported procedures [40] , [50] . Preparation of gold nanoparticles Au- TOASiW9 was prepared as follows: an aqueous solution of HAuCl 4 (20 mL, 5 mM) was mixed with a solution of TOAB in toluene (20 mL, 50 mM). The two-phase mixture was vigorously stirred until all the HAuCl 4 was transferred into the organic layer, and an aqueous solution of NaSiW9 (20 mL, 5 mM) was then added to the organic layer and the resulting solution was stirred for 30 min, followed by a phase-separation to yield the organic layer. A freshly prepared aqueous solution of NaBH 4 (20 mL, 20 mM) was slowly added, and the organic phase was immediately separated and filtrated twice using hydrophobic filters to remove residual water, affording a toluene solution of Au- TOASiW9 . For optimization of TOAB and NaBH 4 usage (Supplementary Table 2 ), the amounts of NaSiW9 and HAuCl 4 were hold constant, and the same procedures were used with the exception of varying the amounts of TOAB and NaBH 4 . Au- TOASiW10 , Au- TOASiW11 , Au- TOASiW12 and Au-TOAB were prepared using similar procedures as that for Au- TOASiW9 , except for using different POMs (K 8 SiW 10 O 36 , K 8 SiW 11 O 39 , K 4 SiW 12 O 40 ) or no POM in the case of Au-TOAB. Gold nanoparticles in other organic solvents were prepared using the same procedures as described for Au- TOASiW9 in toluene but using p -xylene and 1,2-dichloroethane instead of toluene. POM-protected platinum, ruthenium and rhenium nanoparticles (Pt- TOASiW9 , Ru- TOASiW9 , Re- TOASiW9 ) were prepared as described above for Au- TOASiW9 , except for using Na 2 PtCl 6 , K 2 RuCl 5 and K 2 ReCl 6 , respectively, instead of HAuCl 4 . POM-protected rhodium nanoparticles (Rh- TOASiW9 ) was prepared via a slightly modified methodology using RhCl 3 without conducting phase separation until NaBH 4 reduction was complete. Au-dodecanethiol was prepared according to the Brust–Schiffrin method [10] , except by decreasing the concentration for comparison in catalytic test as follows: an aqueous solution of HAuCl 4 (5 mL, 18 mM) was mixed with a solution of TOAB in toluene (20 mL, 20 mM). The two-phase mixture was vigorously stirred until all the HAuCl 4 was transferred into the organic layer, and dodecanethiol (0.9 mmol, 10 equivalents to Au) was then added to the organic phase. A freshly prepared aqueous solution of NaBH 4 (5 mL, 200 mM) was slowly added with vigorous stirring. After further stirring for 3 h, the organic phase was separated and filtrated twice using hydrophobic filters to remove residual water to give a toluene solution of Au-dodecanethiol, that was directly used without further treatment. Titration experiments UV–vis titration procedure, based on changes in SPR absorbance [29] , [30] , was used to quantify the replacement of TOASiW9 by thiolates on the surfaces of the gold nanoparticles. A toluene solution of dodecanethiol (5 mM) was gradually added to a toluene solution of Au- TOASiW9 (0.5 mM Au), and the changes of the absorbance of SPR bands were monitored by UV–vis spectra. The temperature was maintained at 25.0 ± 0.1 °C. Procedure for catalytic reactions The aerobic alcohol oxidation reaction was conducted as follows: 1a (0.25 mmol), biphenyl as an internal standard (0.25 mmol), Au- TOASiW9 (2 mL toluene solution containing 0.01 mmol Au), appended toluene for better dispersion of the base (1 mL) and a magnetic stirrer bar were added to a Pyrex glass reactor, which was then purged with O 2 gas and sealed with a screw cap. The solution was stirred at room temperature (~25 °C) for 24 h. After completion of the reaction, the substrate conversions and product yields were determined via GC analysis. For the reaction under Ar (1 atm), freeze-pump-thaw cycles were carried out and the reactor was connected to a balloon filled with an Ar gas. The oxidative dehydrogenation of piperidone was conducted as follows: 1-methyl-4-piperidone (0.25 mmol), biphenyl as an internal standard (0.25 mmol), Au- TOASiW9 (5 mL toluene solution containing 0.025 mmol Au), and a Teflon-coated magnetic stirrer bar were added to a Pyrex glass reactor, which was purged with O 2 gas and then sealed with a screw cap. The solution was stirred at 70 °C for 24 h. After completion of the reaction, the substrate conversions and product yields were determined via GC analysis. The cross-dehydrogenative coupling reaction of a terminal alkyne and a hydrosilane was conducted as follows: ethynylbenzene (0.25 mmol), triethylsilane (0.3 mmol), biphenyl as an internal standard (0.25 mmol), Au- TOASiW9 (2 mL toluene solution containing 0.01 mmol Au) and a Teflon-coated magnetic stirrer bar were added to a Pyrex glass reactor, which was purged with O 2 gas and sealed with a screw cap. The solution was stirred at 90 °C for 24 h. After completion of the reaction, the substrate conversions and product yields were determined via GC analysis. The regioselective alkynylation of a tertiary amine was conducted as follows: 1-methylpiperidine (0.5 mmol), ethynylbenzene (0.25 mmol), ZnBr 2 (0.25 mmol), biphenyl as an internal standard (0.25 mmol), Au- TOASiW9 (2 mL toluene solution containing 0.01 mmol Au) and a Teflon-coated magnetic stirrer bar were added to a Pyrex glass reactor, which was then purged with O 2 and sealed with a screw cap. The solution was stirred at 90 °C for 24 h. After completion of the reaction, the substrate conversions and product yields were determined via GC analysis. Computational methods First-principles density functional theory calculations were performed by using the CONQUEST code. Double- ζ plus polarization pseudo atomic orbital (PAO) basis functions were used with norm-conserving pseudopotentials. 5 s and 5p semi-core PAOs were used for Au and W. The PAO ranges [bohr] are as follows: Au [5 s, 5p, 5d, 6 s, 6p] = [2.81, 3.36, (7.12, 3.74), (7.12, 3.74), 7.12], Si [3 s, 3p, 3d] = [(7.12, 4.02), (7.12, 4.02), 7.12], W [5 s, 5p, 6 s, 5d, 6p] = [3.22, 3.85, (7.97, 4.18), (7.97, 4.18), 7.97], and O [2 s, 2p, 3d] = [(4.91, 2.58), (4.91, 2.58), 4.91]. The PBE exchange-correlation functional was used. The geometry of SiW9 -protected Au nanoparticle (denoted as Au- SiW9 ) with different orientations was optimised, in which Au was modelled as a nanoparticle of diameter about 2 nm (consisting of 309 atoms) in Oh symmetry. According to the formal charge of SiW9 , we set the charge of the unit cell to be –10 for Au- SiW9 with neutralizing background uniform charge density. The cubic unit cells of 75.6×75.6×75.6 bohr 3 were used for all systems. The grid spacing was 0.21 bohr.